ArabidopsisABCG14 protein controls the acropetal translocation of root-synthesized cytokinins Cytokinins are a major group of phytohormones regulating plant growth, development and stress responses. However, in contrast to the well-defined polar transport of auxins, the molecular basis of cytokinin transport is poorly understood. Here we show that an ATP-binding cassette transporter in Arabidopsis , AtABCG14, is essential for the acropetal (root to shoot) translocation of the root-synthesized cytokinins. AtABCG14 is expressed primarily in the pericycle and stelar cells of roots. Knocking out AtABCG14 strongly impairs the translocation of trans -zeatin ( t Z)-type cytokinins from roots to shoots, thereby affecting the plant’s growth and development. AtABCG14 localizes to the plasma membrane of transformed cells. In planta feeding of C 14 or C 13 -labelled t Z suggests that it acts as an efflux pump and its presence in the cells directly correlates with the transport of the fed cytokinin. Therefore, AtABCG14 is a transporter likely involved in the long-distance translocation of cytokinins in planta. Cytokinins are a heterogeneous class of N 6 -substituted adenine derivatives with either an isoprene-derived or an aromatic side chain [1] , [2] , [3] . Since their discovery in the 1950s as key promoters of cell division in plants, a plethora of biological functions have been attributed to these signalling molecules, encompassing the regulation of cell division and differentiation [4] , chloroplast development [5] , leaf senescence [5] , [6] , root- and shoot-apical dominance [7] , nutrient balances and stress responses [8] . Plants respond to cytokinins through a two-component signalling pathway: cytokinin binding to histidine-kinase receptors induces a phosphorelay that activates two types of response regulators (RRs), and consequently triggers the signal responses [9] . Isoprenoid cytokinins, including trans -zeatin ( t Z), dihydrozeatin (DHZ), cis -zeatin ( c Z) and isopentenyladenine (iP), are the most abundant species in higher plants [1] . Chemical profiling of xylem and phloem sap, and reciprocal grafting of roots and shoots of cytokinin-deficient mutants revealed that t Z-type cytokinins are mainly synthesized in roots, and iP-type cytokinins mainly in shoots. They then, respectively, move acropetally through the xylem and basipetally or systemically through the phloem, and are distributed to the action sites [4] , [10] . Therefore, cytokinins act as both local and long-distance signals in regulating cell division and differentiation. Some in vitro evidence indicates that two types of selective transporter systems may be involved in translocating cytokinin. Members of the Arabidopsis purine permease family, AtPUP1 and PUP2, appear to mediate the import of adenines and nucleobase cytokinins [11] , [12] , while equilibrative nucleoside transporters (ENTs) of both rice and Arabidopsis might mediate the transport of adenosine and other nucleosides, including iP riboside [13] , [14] . However, definitive proof of the involvement of both types of transporters in cytokinin translocation in planta is lacking [9] , [15] . ATP-binding cassette (ABC) transporters comprise one of the largest families of transport proteins, catalysing the export and import of numerous metabolites in organisms ranging from bacteria to humans [16] . The Arabidopsis genome contains more than 120 ABC transporter genes [17] , most of which encode membrane-bound proteins [17] . ABC subfamily G (ABCG) includes 28 members of the white–brown complex half transporters, and 15 pleiotropic drug resistance full transporters [16] . Several members of this subfamily have demonstrated responsibility for exporting wax and cutin used in the formation of cuticle in aerial organs [18] , for conveying abscisic acid across the plasma membrane in leaf guard cells [19] and for exporting auxinic compounds, including indole-3-butyric acid [20] . Seemingly, the ABCG subfamily proteins participate in various biological processes. Nevertheless, although growing numbers of this subfamily of proteins have been characterized, the biological and biochemical functions of many of ABCG proteins remain undetermined. In this study, using a reverse genetics approach to systematically characterize the ABCG proteins, we note that the disruption of AtABCG14 in null mutant lines severely impairs the long-distance translocation and distribution of the root-synthesized t Z-type cytokinin species, which subsequently causes substantial morphological alterations in the growth and development of roots and shoots; furthermore, our in planta feeding and detached leaf assay using a radiolabelled tracer demonstrates an efflux pump activity of AtABCG14 to the fed cytokinin. Therefore, AtABCG14 is a transporter likely involved in the control of acropetal long-distance translocation of t Z-type cytokinins in planta. Disruption of AtABCG14 causes cytokinin-deficient phenotypes Conducting in silico gene expression analysis on a set of Arabidopsis ABCG transporters with unknown function, we found that one of the subfamily members, AtABCG14 , is highly expressed in the vascular tissues of roots. To examine this gene’s function, we obtained two T-DNA insertion mutant alleles, SK_15917 and SK_15918, from Arabidopsis Biological Research Center. By genotyping and reverse transcriptional polymerase chain reaction (RT–PCR) analysis, we verified that both lines with T-DNA insertions in the second exon of the gene are null mutants; we designated them as atabcg14-1 and atabcg14-2 ( Supplementary Fig. 1 ). When grown under normal conditions, both mutant lines exhibited weaker growth, smaller inflorescences and rosettes, slenderer stems and shorter primary roots than their wild-type counterparts ( Fig. 1a–e and Supplementary Fig. 2 ). These morphological alterations are reminiscent of the symptoms of cytokinin deficiency in the cytokinin receptor mutant lines ahk2/ahk3 (ref. 21 ) and in plants overexpressing Arabidopsis CYTOKININ OXIDASE ( AtCKX ) [22] , implying that both mutants might have defective cytokinin signalling pathways or responses. Transformation with a genomic DNA sequence comprising the native AtABCG14 promoter, exons and introns completely restored wild-type morphology in these mutant lines ( Supplementary Fig. 3 ), verifying that AtABCG14 deficiency is the cause of the observed phenotypic deviations. 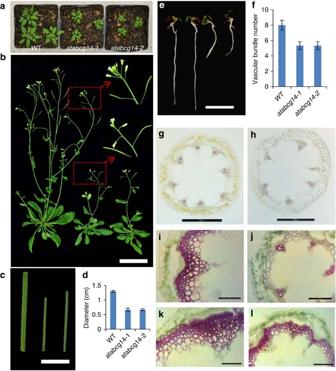Figure 1: Phenotypes ofatabcg14mutants. (a) 25-DAG wild-type (left),atabcg14-1(middle) andatabcg14-2(right) mutant plants. (b) 35-DAG wild-type (left),atabcg14-1(middle) andatabcg14-2(right) mutant plants. Insets show wild-type inflorescences and the smalleratabcg14-1inflorescences ( × 3 magnification). Scale bar, 5 cm. (c) Wild-type (left) and mutant (middle and right) stems. Scale bar, 1 cm. (d) Basal diameter of wild-type andatabcg14mutant stems (means±s.d.,n=8). (e) Root elongation of 8-DAG wild-type (left two),atabcg14-1mutant (third from left) andatabcg14-2mutant (far right) seedlings. Scale bar, 1 cm. (f) Numbers of vascular bundles of wild-type and mutant plants (means±s.d.,n=6). (g) and (h) Phloroglucinol staining of the top parts (below the third generated silique) of wild-type andatabcg14-1mutant inflorescences, respectively, illustrating the reduced numbers of vascular bundles in stems of the mutants. Scale bar, 200 μm. (i) and (j) Phloroglucinol staining of middle part (base of the third internode from the ground) of wild-type andatabcg14-1mutant stems, respectively. (k) and (l) Phloroglucinol staining of basal part (first internode from the ground) of wild-type andatabcg14-1mutant stems, respectively. Scale bars in (i–l), 100 μm. Figure 1: Phenotypes of atabcg14 mutants. ( a ) 25-DAG wild-type (left), atabcg14-1 (middle) and atabcg14-2 (right) mutant plants. ( b ) 35-DAG wild-type (left), atabcg14-1 (middle) and atabcg14-2 (right) mutant plants. Insets show wild-type inflorescences and the smaller atabcg14-1 inflorescences ( × 3 magnification). Scale bar, 5 cm. ( c ) Wild-type (left) and mutant (middle and right) stems. Scale bar, 1 cm. ( d ) Basal diameter of wild-type and atabcg14 mutant stems (means±s.d., n =8). ( e ) Root elongation of 8-DAG wild-type (left two), atabcg14-1 mutant (third from left) and atabcg14-2 mutant (far right) seedlings. Scale bar, 1 cm. ( f ) Numbers of vascular bundles of wild-type and mutant plants (means±s.d., n =6). ( g ) and ( h ) Phloroglucinol staining of the top parts (below the third generated silique) of wild-type and atabcg14-1 mutant inflorescences, respectively, illustrating the reduced numbers of vascular bundles in stems of the mutants. Scale bar, 200 μm. ( i ) and ( j ) Phloroglucinol staining of middle part (base of the third internode from the ground) of wild-type and atabcg14-1 mutant stems, respectively. ( k ) and ( l ) Phloroglucinol staining of basal part (first internode from the ground) of wild-type and atabcg14-1 mutant stems, respectively. Scale bars in ( i – l ), 100 μm. Full size image Atabcg14 mutant seedlings exhibited severe retardation of primary root elongation ( Fig. 1e and Supplementary Fig. 4a,b ). This phenotype is also consistent with perturbation of cytokinin status, as increase in cytokinin levels normally inhibit root growth and reduce the size of root meristems [22] , [23] , [24] . Thus, we speculated that disrupting AtABCG14 may impair root meristem activity. To test this hypothesis, we employed the CYCB1;1::uidA expression cassette, a widely used mitosis reporter [22] , [25] , to monitor meristem activities in the primary roots of Arabidopsis . When the atabcg14-1 mutant was crossed with a CYCB1;1 :: uidA transgenic line, β-glucuronidase (GUS) activity was much weaker in the proximal root meristem of homozygous progeny harbouring the CYCB1;1 :: uidA transgene in an atabcg14-1 mutant background than in CYCB1;1 :: uidA -expressing progeny with a wild-type background ( Supplementary Fig. 4c ). These findings confirm that disrupting AtABCG14 deleteriously affects root meristem activity, possibly by disturbing the concentrations or distribution of root cytokinins. Further, we monitored the responses of root elongation of atabcg14 plants to phytohormones and hormone precursors at various concentrations, including the ethylene precursor 1-aminocyclopropane-1-carboxylic acid (ACC), the auxin 1-naphthaleneacetic acid (NAA) and the cytokinins 6-benzyladenine (BA) and t Z. Exogenously applying these substances to vertically growing seedlings generally inhibited root elongation in a dose-dependent manner ( Supplementary Fig. 5 ). However, root elongation was distinctly less sensitive to BA and t Z treatments in atabcg14 mutants than in wild-type plants. In sharp contrast, responses of the mutant and wild-type plants to exposure to auxin and ACC were indistinguishable ( Supplementary Fig. 5 ). These data further imply that in mutant roots there may be a change in endogenous cytokinin homeostasis or cytokinin-related signalling perception or response. Consistent with having slender inflorescence stems, the average number of vascular bundles was reduced considerably in the atabcg14 mutant lines, from 8±0.63 (mean±s.d., n =6) in wild-type plants to about 5.3±0.52 (mean±s.d., n =6) ( Fig. 1f–h ). This affords us anatomical evidence of cytokinin perturbation in the mutant lines, because, as well as regulating root meristems, cytokinins are key regulators of shoot meristem activity, but in an opposite manner [22] , [26] . Cytokinin deficiencies reportedly diminish the activities of vegetative and floral shoot meristems, including cambium-mediated secondary growth [4] , [22] , [26] . Furthermore, the numbers of cells in phloem and xylem in the vascular bundle were reduced; lignin synthesis and deposition (key processes in cell differentiation and secondary cell wall thickening) were considerably delayed, and the numbers of lignified cells were substantially reduced in the interfascicular fibres and xylem bundles of the mutant plants ( Fig. 1i–l ). This syndrome largely resembles secondary growth retardation observed in the atipt1;3;5;7 quadruple mutant, where the key genes encoding ATP/ADP:isopentenyltransferases ( IPTs) responsible for synthesizing cytokinins are disrupted, leading to low levels of cytokinins and reducing cambial activity in the shoot [4] . The altered secondary thickening of the atabcg14 mutant points to a decline in fascicular- and interfascicular-cambial activity, implying a potential shortage of cytokinins in atabcg14 shoots. Besides the shorter primary roots and slender inflorescence stems, the mutant seedlings had shorter leaf petioles, smaller leaf areas and about 40% lower chlorophyll a and b contents than did wild-type plants, and thus were pale yellow rather than green ( Supplementary Fig. 6 ). This is consistent with cytokinins’ well-documented role in promoting chlorophyll retention [5] , [21] , and further implies that atabcg14 mutants have cytokinin deficiencies in their aerial tissues. Thus, the morphological, anatomical and physiological data collectively imply that disrupting AtABCG14 interferes with the distribution and/or concentrations of cytokinins in both roots and shoots. atabcg14 impairs the acropetal distribution of cytokinins To verify whether AtABCG14 participates in controlling cytokinin distribution in planta , we monitored GUS expression, driven by Arabidopsis RR 5 promoter ( ARR5::GUS ), in the atabcg14 mutant lines. ARR5 is a type-A cytokinin RR gene of the two-component system that is transcriptionally upregulated by cytokinins. Thus, changes in the concentrations of endogenous cytokinins affect its expression [22] , [27] . For demonstrating this, we crossed atabcg14 with ARR5::GUS transformants and then examined GUS activity in seedlings of the homozygous cross-progenies (6 days after germination, 6-DAG). The progeny seedlings showed similar retardation in growth and losses in chlorophyll to the atabcg14 mutant ( Fig. 2a,b ). The spatial expression patterns of GUS in the shoots and roots of ARR5::GUS / atabcg14 seedlings sharply differed from those in ARR5::GUS /WT plants ( Fig. 2c,d ). In the wild-type background, GUS was abundantly expressed in the shoot/cotyledon leaves, and weakly expressed in the root cap’s statocytes and the upward vascular cylinder. In contrast, GUS activity was diminished by 71% in cotyledon leaves of ARR5::GUS / atabcg14 seedlings, but strongly increased (about threefold) in their primary roots ( Fig. 2e ), where the GUS signals were widely distributed across all the cell types, including the cells of the epidermis, cortex and endoderm ( Fig. 2d ). These data clearly indicate that there are opposite patterns of cytokinin distribution in the roots and shoots of atabcg14 and wild-type plants, and that cytokinin levels were low in shoots but high in roots of the mutants ( Fig. 2e ). Similarly, in the inflorescences of mature plants, GUS activity was substantially weaker in ARR5 :: GUS / atabcg14 than in ARR5 :: GUS /WT plants ( Fig. 2f ). The GUS signals were clearly visible in the stigma, anther and receptacle of ARR5 :: GUS /WT plants, but undetectable in those of ARR5 :: GUS / atabcg14 plants ( Supplementary Fig. 7 ). The altered spatial expression of ARR5::GUS in the atabcg14 background strongly suggests that disruption of AtABCG14 impairs the allocation of cytokinins between roots and shoots. 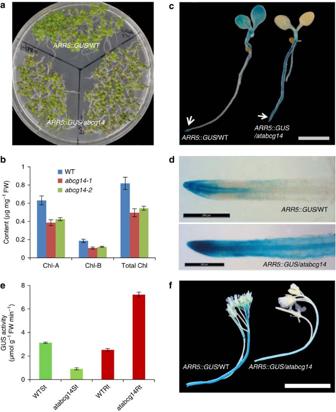Figure 2: Expression ofARR5::GUSreporter inatabcg14mutants. (a) Photograph illustrating phenotypes of 6-DAGARR5::GUS/WT andARR5::GUS/atabcg14seedlings. (b) Chlorophyll contents in 6-DAGARR5::GUS/WT andARR5::GUS/atabcg14seedlings. WT representsARR5::GUS/WT;atabcg1-1and-2representARR5::GUS/atabcg14lines1and2, respectively. Chl-A, Chl-B and Total Chl represent chlorophyll a, chlorophyll b and total chlorophyll contents, respectively (means±s.e.,n=4). (c) GUS staining (6 h) ofARR5::GUS/WT (left) andARR5::GUS/atabcg14(right) seedlings. Note the distinct distribution of GUS signal in the shoot and root of wild-type andatabcg14plants. Arrows indicate the GUS staining in root tips. Scale bar, 0.5 cm. (d) Close-up of the portion of primary roots ofARR5::GUS/WT andARR5::GUS/atabcg14plants arrowed in (c). Scale bars, 200 μm. (e) GUS activity (means±s.e.,n=3) in shoots and roots of 8-DAGARR5::GUS/WT andARR5::GUS/atabcg14seedlings. St, shoot; Rt, root. (f) GUS staining (12 h) ofARR5::GUS/WT andARR5::GUS/atabcg14inflorescences. Scale bar, 1 cm. Figure 2: Expression of ARR5::GUS reporter in atabcg14 mutants. ( a ) Photograph illustrating phenotypes of 6-DAG ARR5::GUS/ WT and ARR5::GUS / atabcg14 seedlings. ( b ) Chlorophyll contents in 6-DAG ARR5::GUS /WT and ARR5::GUS / atabcg14 seedlings. WT represents ARR5::GUS /WT; atabcg1-1 and -2 represent ARR5::GUS / atabcg14 lines 1 and 2 , respectively. Chl-A, Chl-B and Total Chl represent chlorophyll a, chlorophyll b and total chlorophyll contents, respectively (means±s.e., n =4). ( c ) GUS staining (6 h) of ARR5::GUS /WT (left) and ARR5::GUS / atabcg14 (right) seedlings. Note the distinct distribution of GUS signal in the shoot and root of wild-type and atabcg14 plants. Arrows indicate the GUS staining in root tips. Scale bar, 0.5 cm. ( d ) Close-up of the portion of primary roots of ARR5::GUS /WT and ARR5::GUS / atabcg14 plants arrowed in ( c ). Scale bars, 200 μm. ( e ) GUS activity (means±s.e., n =3) in shoots and roots of 8-DAG ARR5::GUS /WT and ARR5::GUS / atabcg14 seedlings. St, shoot; Rt, root. ( f ) GUS staining (12 h) of ARR5::GUS /WT and ARR5::GUS / atabcg14 inflorescences. Scale bar, 1 cm. Full size image Altered distribution of t Z-type cytokinins in atabcg14 t Z-type cytokinins primarily are synthesized in the root and translocated to the shoot via the xylem flow [4] . Profiling the cytokinin species of atabcg14 mutants by LC-MS/MS revealed fivefold reductions in the total levels of t Z-type cytokinins in their shoots, with corresponding increase in their roots, compared with wild-type controls ( Table 1 and Supplementary Table 1 ). Particularly, t Z N 7 -glucoside, the major storage form of t Z-type cytokinins in Arabidopsis , was reduced to <20% of wild-type levels in atabcg14 shoots, but were more than fourfold higher in the roots ( Supplementary Table 1 ). In addition, the contents of DHZ-type cytokinins (metabolically derived from t Z precursors) were more than 62% lower than wild-type levels in shoots, with concomitant increases (up to tenfold) in the roots of the atabcg14 mutants. These data demonstrate that knocking out AtABCG14 impairs the distribution of the root-synthesized t Z- and DHZ-type cytokinins in root and shoot. In contrast to the decline of both t Z- and DHZ-type cytokinins in the mutant shoots, the iP-type cytokinins (known to be synthesized in the shoots and transported via phloem flow) were increased in both the shoots and roots, as were the c Z-types that are synthesized from isopentenylated RNAs [28] ( Table 1 ). This implicates an intrinsic homeostatic mechanism that plant cells may take to compensate for perturbations in synthesis and distribution of different types of cytokinins. Overall, these data indicate that AtABCG14 plays a key role in distribution of the root-synthesized t Z- or DHZ-type cytokinins in planta . Table 1 Total cytokinin levels in shoots and roots of wild-type and atabcg14 mutant plants. Full size table AtABCG14 expression in root pericycle and stelar cells To further assess the function of AtABCG14 in planta , we investigated its expression pattern by using the 1.3-kb region 5′-upstream of the gene to drive expression of GUS or the enhanced green fluorescent protein ( EGFP ) -AtABCG14 fusion cassette. Expression of the latter morphologically complemented the mutant phenotype ( Supplementary Fig. 8 ), indicating that the selected upstream sequence represents a functional promoter and the EGFP-AtABCG14 fusion functions in planta . In 4-DAG seedlings, strong green fluorescent protein (GFP) signals appeared in the root and very weak signals in the shoot ( Fig. 3a ). In the primary root, GFP signals were primarily located in the pericycle and stelar cells ( Fig. 3b,c ). When examining AtABCG14::GUS expression in young seedling, the GUS staining was mainly detected in the transition and elongation/differentiation zones of the primary root, but was absent from its division zone ( Fig. 3d ). These findings are consistent with the reported spatial distribution and functional sites of cytokinins in roots [29] . Consistently, in the transition and elongation/differentiation zones, GUS signals were also mainly detected in the pericycle and stelar cells ( Fig. 3e ). In plants approaching the bolting stage (25-DAG), AtABCG14 was moderately expressed in the young rosette leaves in addition to the roots, especially in the midribs and veins ( Fig. 3f,g ). In the reproductive stage, AtABCG14::GUS expression was also detected in the open flowers, particularly in the mature anthers, and in siliques ( Fig. 3h–j ). Quantitative RT–PCR (qRT–PCR) analysis of 35-DAG plants in the reproductive stage showed that AtABCG14 transcripts were mainly present in the root and inflorescence ( Fig. 3k ). 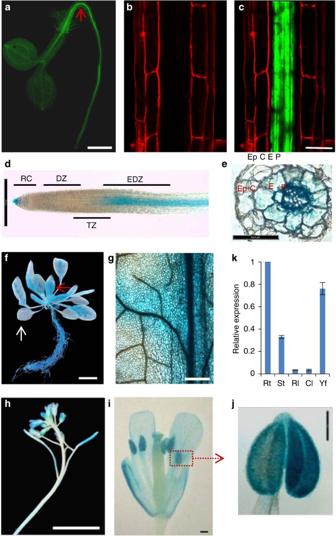Figure 3: Gene expression pattern and subcellular localization of AtABCG14. (a) Distribution of GFP signals in a 4-DAGAtABCG14::EGFP-ABCG14transgenic seedling. Arrow indicates the primary expression in roots. Scale bar, 500 μm. (b) and (c) PI staining ofAtABCG14::EGFP-ABCG14transgenic roots (b) and merged image with GFP signal (c) observed under a confocal microscope, showing expression ofAtABCG14in the pericycle and stelar cells in roots of (a). Scale bar, 25 μm. (d) GUS staining (6 h) in the root of aAtABCG14::GUStransgenic plant. RC, root cap; DZ, division zone; TZ, transition zone; and EDZ, elongation/differentiation zone. Scale bar, 200 μm. (e) Cross-section of the elongation zone of the primary root of anAtABCG14::GUStransgenic plant. Ep, epidermis; C, cortex; E, endodermis; P, pericycle. Scale bar, 50 μm. (f) GUS staining (12 h) of a 25-DAGAtABCG14::GUStransgenic plant. White and red arrows indicate an old leaf and a young, actively growing leaf, respectively. Scale bar, 1 cm. (g) The enlarged image of a GUS-staining leaf. Scale bar, 500 μm. (h) GUS staining (12 h) in the young inflorescence of anAtABCG14::GUStransgenic plant. Scale bar, 1 cm. (i) GUS staining (12 h) in the open flower of anAtABCG14::GUStransgenic plant. Scale bar, 100 μm. (j) GUS staining (12 h) in the mature anther from (i). Scale bar, 100 μm. (k) qRT–PCR analysis ofAtABCG14expression in 35-DAG plants. Rt, root; St, stem; RL, rosette leaves; CL, cauline leaves; Yf, young inflorescence. TheACTIN 2gene was used as the control. Data are means±s.e. (n=3). Figure 3: Gene expression pattern and subcellular localization of AtABCG14. ( a ) Distribution of GFP signals in a 4-DAG AtABCG14::EGFP-ABCG14 transgenic seedling. Arrow indicates the primary expression in roots. Scale bar, 500 μm. ( b ) and ( c ) PI staining of AtABCG14::EGFP-ABCG14 transgenic roots ( b ) and merged image with GFP signal ( c ) observed under a confocal microscope, showing expression of AtABCG14 in the pericycle and stelar cells in roots of ( a ). Scale bar, 25 μm. ( d ) GUS staining (6 h) in the root of a AtABCG14::GUS transgenic plant. RC, root cap; DZ, division zone; TZ, transition zone; and EDZ, elongation/differentiation zone. Scale bar, 200 μm. ( e ) Cross-section of the elongation zone of the primary root of an AtABCG14::GUS transgenic plant. Ep, epidermis; C, cortex; E, endodermis; P, pericycle. Scale bar, 50 μm. ( f ) GUS staining (12 h) of a 25-DAG AtABCG14::GUS transgenic plant. White and red arrows indicate an old leaf and a young, actively growing leaf, respectively. Scale bar, 1 cm. ( g ) The enlarged image of a GUS-staining leaf. Scale bar, 500 μm. ( h ) GUS staining (12 h) in the young inflorescence of an AtABCG14::GUS transgenic plant. Scale bar, 1 cm. ( i ) GUS staining (12 h) in the open flower of an AtABCG14::GUS transgenic plant. Scale bar, 100 μm. ( j ) GUS staining (12 h) in the mature anther from ( i ). Scale bar, 100 μm. ( k ) qRT–PCR analysis of AtABCG14 expression in 35-DAG plants. Rt, root; St, stem; RL, rosette leaves; CL, cauline leaves; Yf, young inflorescence. The ACTIN 2 gene was used as the control. Data are means±s.e. ( n =3). Full size image AtABCG14 localizes on the plasma membrane So far, all the characterized ABCG proteins, except ABCG19, were localized to plasma membrane [30] . To probe the subcellular localization of AtABCG14, we transiently expressed the 35S::EGFP-AtABCG14 chimeric cassette in Arabidopsis leaf protoplasts. We noted that the fluorescence signals of the fusion protein primarily appeared in the rims of the protoplasts, just outside the clumps of chloroplasts that were located in the corner of cytoplasm ( Fig. 4a ). In sharp contrast, the free GFP expressed in the protoplasts appeared to be widely distributed inside the inner protoplast membrane, while the chloroplasts were dispersed within the fluorescent region ( Fig. 4b ). When the 35S::EGFP-AtABCG14 cassette was stably expressed in the atabcg14 mutants, they were phenotypically rescued ( Supplementary Fig. 9a ). The fluorescence distribution of the fusion protein in leaf epidermal cells agreed well with that revealed by FM4-64 staining, a typical plasma membrane indicator [31] , and also lined up with the adjacent cell wall that was labelled with propidium iodide (PI), the cell wall polysaccharide indicator [31] ( Fig. 4c,d ). Further, when we subjected the leaf cells to plasmolysis, the GFP signal co-segregated with FM4-64 staining ( Supplementary Fig. 9b ), whereas the GFP signal and PI staining separated when the leaf cells were similarly treated ( Supplementary Fig. 9c ). To further confirm AtABCG14’s subcellular localization, we purified the plasma membrane fraction from Arabidopsis seedlings stably transformed with 35S::EGFP-AtABCG14 using an aqueous-polymer two-phase partitioning procedure [32] . Immunoblots with anti-GFP antibody revealed that the EGFP-AtABCG14 fusion dominated in plasma membrane preparation (upper phase), where the plasma membrane marker H + -ATPase coexists ( Fig. 4e and Supplementary Fig. 10 ). These microscopic observations and gel-blot analyses indicate that AtABCG14 is a plasma membrane-localized protein. 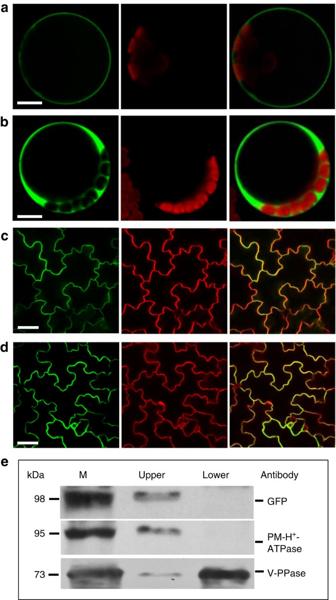Figure 4: Subcellular localization of EGFP-AtABCG14 fusion protein. (a) and (b) Fluorescence distribution when35S::EGFP-AtABCG14(a) or35S::EGFP(b) was expressed in tobacco leaf protoplasts (left); autoflorescence of chloroplasts and merged images are shown in the middle and right, respectively. Scale bar, 5 μm. (c) Distribution of EGFP-AtABCG14 fluorescence in leaf epidermal cells (left), FM4-64 staining (middle) and merged image (right). Scale bar, 5 μm. (d) Distribution of EGFP-AtABCG14 fluorescence in rosette leaf epidermal cells (left), PI staining (middle) and merged image (right). Scale bar, 5 μm. (e) Immunoblot analysis of membrane fractions from EGFP-AtABCG14 expressing seedlings by probing with antibodies against GFP,Arabidopsisplasma membrane H+-ATPase (PM-H+-ATPase) and vacuolar H+-pyrophosphatase (V-PPase, tonoplast marker). Figure 4: Subcellular localization of EGFP-AtABCG14 fusion protein. ( a ) and ( b ) Fluorescence distribution when 35S::EGFP-AtABCG14 ( a ) or 35S::EGFP ( b ) was expressed in tobacco leaf protoplasts (left); autoflorescence of chloroplasts and merged images are shown in the middle and right, respectively. Scale bar, 5 μm. ( c ) Distribution of EGFP-AtABCG14 fluorescence in leaf epidermal cells (left), FM4-64 staining (middle) and merged image (right). Scale bar, 5 μm. ( d ) Distribution of EGFP-AtABCG14 fluorescence in rosette leaf epidermal cells (left), PI staining (middle) and merged image (right). Scale bar, 5 μm. ( e ) Immunoblot analysis of membrane fractions from EGFP-AtABCG14 expressing seedlings by probing with antibodies against GFP, Arabidopsis plasma membrane H + -ATPase (PM-H + -ATPase) and vacuolar H + -pyrophosphatase (V-PPase, tonoplast marker). Full size image AtABCG14 transports the C 14 -t Z tracer To explore the involvement of AtABCG14 in translocating t Z-type cytokinins, we fed C 14 -labelled t Z to the roots of wild-type and atabcg14 mutant seedlings. We subsequently detected strong radioactivity in the shoots of wild-type plants, but only trace amounts in the mutants’ shoots ( Fig. 5a ). However, radioactivity was enriched in their roots ( Fig. 5b ). In contrast, when S-adenosyl- L -C 14 -methionine was fed to the seedlings, as the control, it was effectively conveyed from the roots to shoots in both wild-type and mutant plants, and there was no clear difference in the distributions of radioactivity ( Fig. 5c,d ). Furthermore, when C 14 - t Z was fed to the functional complementary lines ( atabcg14 mutants harbouring the AtABCG14::EGFP-AtABCG14 cassette), the transport of C 14 - t Z to the shoots was not only completely restored but was about 2.5-fold higher than in wild-type plants ( Fig. 5e ). qRT–PCR analysis revealed that the expression level of AtABCG14 in this complementary line was about sixfold higher than in the wild type ( Fig. 5f ), presumably due to the presence of multiple copies of the expression cassette. These data demonstrate a direct correlation between C 14 - t Z transport activity and the expression level of AtABCG14. Furthermore, when both wild-type and mutant seedlings were fed with C 14 - t Z for a series of time periods, the radioactivity progressively accumulated in the wild-type shoots, whereas none or only negligible amounts of activity was detected in those mutant lines over 5 h, a finding that further suggests that a deficiency of AtABCG14 abolishes the translocation of C 14 - t Z from root to shoot ( Fig. 5g ). To ascertain whether the radioactivity detected in the fed seedlings represents t Z or its derivatives, we fed the stable isotope tracer C 13 - t Z to the roots of both wild-type and mutant seedlings, and monitored its translocation and potential transformation by LC-MS. Over a 4-h incubation period, the detected C 13 labels in shoots predominantly either were the original form of C 13 - t Z or its natural derivatives such as the riboside, and O / N -glycoside, and they were accumulated in wild-type shoots but nearly undetectable in the mutant shoots ( Table 2 ). Collectively, these data confirm the involvement of AtABCG14 in t Z-type cytokinin transport from root to shoot in planta. 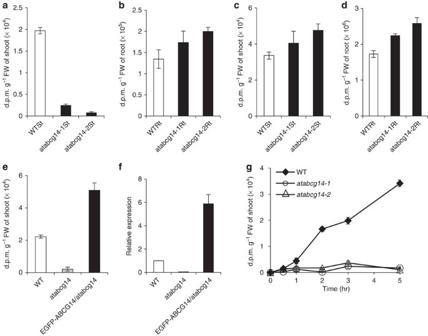Figure 5: Effect of AtABCG14 on translocation of cytokinin from root to shoot. Radioactivity in the following organs of wild-type andatabcg14mutant seedlings: (a) shoots (St) after feeding C14-tZ to their roots (Rt); (b)roots after feeding C14-tZ to their roots; (c) shoots after feeding S-adenosyl-L-C14-methionine (C14-SAM) to their roots; (d) roots after feeding C14-SAM to their roots. (e) Radioactivity in shoots of wild-type,atabcg14and seedlings harbouringAtABCG14::EGFP-AtABCG14cassette after feeding C14-tZ to their roots; (f) the relative expression levels of theAtABCG14in wild-type,atabcg14and seedlings harbouringAtABCG14::EGFP-AtABCG14cassette. TheUBIQUITIN 10gene was used as the control. Data are means±s.d. (n=3); (g) radioactivity in shoots of wild-type andatabcg14mutant seedlings after feeding C14-tZ to their roots in a time course. Data in (a–e) and in (g) are means±s.e. (n=3). Figure 5: Effect of AtABCG14 on translocation of cytokinin from root to shoot. Radioactivity in the following organs of wild-type and atabcg14 mutant seedlings: ( a ) shoots (St) after feeding C 14 - t Z to their roots (Rt); ( b )roots after feeding C 14 - t Z to their roots; ( c ) shoots after feeding S-adenosyl- L -C 14 -methionine (C 14 -SAM) to their roots; ( d ) roots after feeding C 14 -SAM to their roots. ( e ) Radioactivity in shoots of wild-type, atabcg14 and seedlings harbouring AtABCG14::EGFP-AtABCG14 cassette after feeding C 14 - t Z to their roots; ( f ) the relative expression levels of the AtABCG14 in wild-type, atabcg14 and seedlings harbouring AtABCG14::EGFP-AtABCG14 cassette. The UBIQUITIN 10 gene was used as the control. Data are means±s.d. ( n =3); ( g ) radioactivity in shoots of wild-type and atabcg14 mutant seedlings after feeding C 14 - t Z to their roots in a time course. Data in ( a – e ) and in ( g ) are means±s.e. ( n =3). Full size image Table 2 The detected C 13 -labelled species in shoots and roots of wild-type and atabcg14 mutant fed with C 13 - t Z. Full size table ABC transporters can function either as importers or exporters [16] . Thus, to further investigate the direction of ABCG14-mediated transport of cytokinins, we incubated detached leaves from 12-DAG transgenic seedlings harbouring 35S::EGFP-AtABCG14 ( Supplementary Fig. 9a ) with C 14 - t Z, followed by a thorough wash; we then detected the remaining radioactivity in leaf cells. In plants harbouring 35S::EGFP-AtABCG14 , AtABCG14 was expected to be expressed ectopically in all types of cells, including the leaf epidermis as shown by the GFP fluorescence distribution ( Fig. 4c,d ), whereas the expression of ABCG14 in wild-type leaves was weak, and restricted to the vein cells ( Fig. 3a,f and g ). Indeed, qRT–PCR showed that the transcript level of AtABCG14 is more than 250-fold higher in the detached leaves of overexpression lines than in wild-type control ( Fig. 6a ). Accordingly, the accumulated C 14 -radioactivity in leaf cells of the transgenic plants was four times lower than in wild-type controls ( Fig. 6b ). In contrast, the uptake of C 14 -SAM did not markedly differ between transgenic and wild-type leaves ( Fig. 6c ). Moreover, pre-treatment of the detached leaves with the specific inhibitor of the ABC type transporter, sodium ortho -vanadate, substantially mitigated the loss of radioactivity in the cells harbouring 35S::EGFP-AtABCG14 ( Fig. 6b ). Furthermore, throughout the incubation period with C 14 - t Z, the difference in the accumulated radioactivity between wild-type and transgenic leaf cells remained constant ( Fig. 6d ).These data corroborate that the less uptake of the transgenic leaf cells to the fed radiotracer is attributed to AtABCG14 activity and that AtABCG14 likely functions as an exporter for the fed tracer. 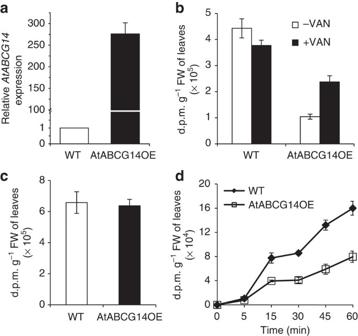Figure 6: AtABCG14 cytokinin (trans-zeatin) transport activity. (a) The relative expression levels of theAtABCG14in the leaves of wild type and an overexpression line harbouring35S::EGFP-AtABCG14(AtABCG14OE). TheUBIQUITIN 10gene was used as the control. Data are means±s.d. (n=3). (b) Radioactivity in the detached leaves of wild-type plants and overexpression line after feeding with C14-tZ in the presence or absence of 1 mM sodium vanadata for 1 h. (c) Radioactivity in the detached leaves of wild-type plants and overexpression line after feeding with C14-SAM. (d) Radioactivity in the detached leaves of wild-type plants and overexpression line after feeding with C14-tZ over a time course. Data in (b–d) are means±s.e. (n=3). Figure 6: AtABCG14 cytokinin ( trans -zeatin) transport activity. ( a ) The relative expression levels of the AtABCG14 in the leaves of wild type and an overexpression line harbouring 35S::EGFP-AtABCG14 (AtABCG14OE). The UBIQUITIN 10 gene was used as the control. Data are means±s.d. ( n =3). ( b ) Radioactivity in the detached leaves of wild-type plants and overexpression line after feeding with C 14 - t Z in the presence or absence of 1 mM sodium vanadata for 1 h. ( c ) Radioactivity in the detached leaves of wild-type plants and overexpression line after feeding with C 14 -SAM. ( d ) Radioactivity in the detached leaves of wild-type plants and overexpression line after feeding with C 14 - t Z over a time course. Data in ( b – d ) are means±s.e. ( n =3). Full size image Cytokinins can act as autocrine, paracrine or long-distance signals [1] , [10] , and different types of cytokinins are synthesized and distributed in distinct tissues or cell types. Several cytokinin biosynthetic genes are found mainly expressed in the root, for instance, AtIPT1 and AtIPT7 are primarily expressed in the vascular stele of the elongation zone and/or root phloem companion cells, indicating that these sites are major sources of root-derived cytokinins [33] . Moreover, the xylem sap of several plant species predominantly contains t Z-type cytokinins, especially t Z riboside ( t ZR) [10] , [34] . These data suggest that the roots, particularly the root pericycle and phloem company cells, are the main sites of t Z production and that t ZR might act as an acropetal signal. In contrast, iP- and c Z-types are the main cytokinins in phloem sap, where they might function as basipetal or systemic signals [10] , [33] , [34] . Members of the purine permease family [11] , [12] and ENT family [10] , [14] hypothetically are involved in cytokinin transport. One of the former, AtPUP1, is reportedly expressed in the epithelium of hydathodes, and the stigma surface, suggesting a potential role in retrieving cytokinins from xylem sap, thus preventing losses during guttation, while AtPUP2 is expressed mainly in phloem, implying a role in long-distance transport of phloem cytokinins [11] , [12] . The ENT transporters putatively mediate translocation of adenosine and other nucleosides, including iPR and t ZR [10] , [14] . Both of these types of transporters were implicated to be involved (based on in vitro data), as cytokinin importers, in the maintenance of either nucleobase homeostasis, or the phloem flow of cytokinins. However, definitive in planta proof is lacking of their role in cytokinin transport. Several lines of evidence obtained in the present study strongly indicate that AtABCG14, a previously uncharacterized half-molecule ABC family member, plays a pivotal role in the long-distance translocation of root-synthesized t Z- and DHZ-type cytokinins in Arabidopsis . This evidence includes the following: the morphological and physiological perturbations exhibited in the atabcg14 mutant alleles, the predominant pericycle gene expression pattern of AtABCG14 , the plasma membrane localization of the encoded protein, the disturbed distribution of cytokinins in roots and shoots of the atabcg14 null mutants and the close correlation of the translocation of exogenously supplied C 14 - t Z with the activity of AtABCG14. In particular, knocking out AtABCG14 almost completely diminished the translocation of the fed radio-tracers from the root to shoot over the entire incubation period, while the complementation of gene expression completely restored their transport ( Fig. 5 ). Moreover, the root-to-shoot transport activity to C 14 - t Z is closely proportionate to the levels of AtABC14 expression in the wild-type, mutant and complementary (or overexpression) lines ( Figs 5 and 6 ). Finally and more definitively, the transport assays using detached leaves showed that transgenic cells with high-level constitutive expression of AtABCG14 exhibited significant efflux activity to the fed C 14 - t Z, and that such activity was sensitive to the application of sodium vanadate, the specific ABC transporter inhibitor ( Fig. 6 ); together, these findings substantiate the involvement of AtABCG14 in transporting t Z-type cytokinins. Therefore, ABC transporters represent a novel family of transporters for cytokinin compartmentalization in planta . The exact transporting form of t Z-type cytokinins mediated by the action of AtABCG14 remains undetermined. Our attempt to determine AtABCG14’s biochemical properties in vitro was unsuccessful. This is probably due to the assay systems that we adopted were not optimal for the effective functional detection or due to the transporter’s half-molecular nature and the possible requirement for an unknown hetero-partner for its proper functioning [31] . These technical obstacles currently prevented our unequivocal assessment of its biochemical function; nevertheless, our transport activity assay using detached leaves, in which one set of leaf cells, as the control, was from a wild-type background that showed very low level of (or even negligible) expression of AtABCG14, and the other set of leaves harboured the overexpressed AtABCG14 (about 250-fold higher in its transcripts, compared with the control leaves), does closely resemble a conventional in vitro assay system for examining this transporter’s function. In addition, monitoring the fed stable isotope in seedlings by LC-MS clearly links the translocation of the fed t Z (and its derivatives) with the necessity of existence of AtABCG14 in cells ( Table 2 ). Therefore, our comprehensive C 14 and C 13 tracer feeding experiments in planta and our ‘semi’- in vitro transport assay using detached leaves provided essential genetic and biochemical evidence showing that AtABCG14, as an exporter, likely functions in transporting/distributing t Z-type cytokinin species. The promoter of AtABCG14 drove GFP or GUS expression in the root’s pericycle and stelar cells ( Fig. 3b,c,e ). This finding is reminiscent of the expression pattern of the BOR1 exporter that is predominantly expressed in the root’s pericycle cells and is responsible for xylem loading of boric acid [35] . Therefore, the presence of AtABCG14, as an efflux pump therein, most likely is involved in transferring root-synthesized cytokinins into the xylem for their long-distance translocation. Besides the predominant expression in the pericycle and stelar cells of the root-elongation zone, like many other genes involved in cytokinin biosynthesis, AtABCG14 was also expressed in inflorescence/open flowers, siliques and the young leaves. Its precise physiological functions in these tissues are still unknown. However, as an efflux pump, the presence of AtABCG14 in diverse tissues implies that it may also participate in the paracrine (transcellular) transport of cytokinins to the apoplast or neighbouring cells, in addition to xylem loading in the roots. Interestingly, root elongation in atabcg14 mutants is less sensitive to exogenous cytokinins than that it is in wild-type plants ( Supplementary Fig. 5 ). Although this characteristic phenotypically resembles the behaviour of cytokinin receptor mutant line cre1/ahk4 , in which the perception of cytokinin signals is defective in the root [36] , mechanistically it may be quite distinct. One possible explanation is that the already high abundance of cytokinins in roots of atabcg14 mutants, resulting from the defect in root-to-shoot translocation ( Table 1 ), may compromise the sensitivity of the root meristem cells in perceiving the exogenously applied signal molecules. Further study is needed to clarify this. We believe that the presented findings have important practical implications. Cytokinins delay leaf senescence, thereby extending the photosynthetic period [5] , [6] , [21] and enhancing the plant’s photosynthate production capacities. They also play key roles in regulating reproductive development and sink strength [37] , [38] ; thus, they are among the most important target hormones for improving crop yields. Furthermore, they are pivotal signals in communicating nitrogen availability from roots to shoots via the xylem vessels [10] , [33] . However, the regulation of their distribution in plants is poorly understood. We identified and characterized AtABCG14 as a key player in the long-distance transport of cytokinins, particularly t Z (the commonest cytokinin in higher plants, and highly active in receptor assays and bioassays [39] ). This finding will provide insight into the molecular mechanisms involved in cytokinin partitioning. Moreover, the results may open new avenues for modifying various important crops, agriculturally, biotechnologically and horticulturally, to increase yields and reduce fertilizer requirements for instance, while improving the exploitation of sustainable bioenergy resources. Plant materials and growth conditions Arabidopsis thaliana ecotype Columbia was used as the wild type for all experiments. The T-DNA insertion lines SK_15917 and SK_15918 were obtained from the Arabidopsis Biological Resource Center. ARR5::GUS and CYCB1;1 :: uidA transgenic seeds were kindly provided by Drs Thomas Schmülling (Free University of Berlin) and Peter Doerner (University of Edinburgh), respectively. Seeds were sown on petri dishes containing half-strength MS with 0.25% phytogel or 0.7% w/v phytoagar and appropriate antibiotics, then kept at 4 °C for 3 days before being moved to a growth chamber. Seedlings with two true leaves were transplanted into soils. Wild-type, mutant and/or transgenic plants were grown side by side in the same tray to minimize possible variations in growth conditions. Plants were grown at 22 °C in a growth chamber under a long-day regime (16-h light/8-h dark) unless otherwise stated. The seedling root elongation assay was performed in a growth chamber at 22 °C under a 14-h light/10-h dark regime. Identification of T-DNA insertion atabcg14 null mutants The T-DNA specific primer pSKTAIL-L1 and the gene-specific primers ABCG14-P1 and ABCG14-P2 were used to identify homozygous atabcg14 mutants at genomic DNA and transcriptional levels, respectively. All primers used in this study are listed in Supplementary Table 2 . Phenotyping and histochemical analysis The diameter of the basal primary stem was measured using a Vernier caliper. Histochemical analysis was performed using 30-μm-thick sections from stems at the same position of wild-type and atabcg14 mutants following the standard protocols of phloroglucinol staining [40] . The number of vascular bundle was calculated based on the observation from the young (top) stems. Vector construction The coding region of the AtABCG14 gene amplified by primers ABCG14-P3 and ABCG14-P4 was cloned into gateway entry vector pDONR207 to form pDONR207-ABCG14 via BP reaction. To construct 35S::ABCG14 and 35S::GFP-ABCG14 binary vectors, the AtABCG14 in pDONR207-AtABCG14 was introduced into pMDC32 and pMDC43, respectively, via LR reactions. To make 35S::EGFP-ABCG14 and AtABCG14::EGFP-ABCG14 constructs, the ABCG14 coding region was amplified by primers ABCG14-P5 and ABCG14-P6 then cloned into the EGFP vector of pSAT6-GFP-N1 (ref. 41 ) at the EcoRI and BamHI restriction sites to form pSAT6-35S::EGFP-ABCG14. The 35S promoter of pSAT6-35S::EGFP-AtABCG14 was then replaced by the AtABCG14 promoter amplified by ABCG14-P7 and ABCG14-P8 from genomic DNA at AgeI and NcoI sites to form the shuttle vector pSAT6-AtABCG14::EGFP-ABCG14. 35S::EGFP-ABCG14 and ABCG14::E GFP-AtABCG14 expression cassettes were released from the pSAT6 shuttle vectors with PI-PspI, and subcloned into the binary vector pPZP-RCS2 to form binary vectors pPZP-35S::EGFP-ABCG14 and pPZP -ABCG14::EGFP-ABCG14, respectively. To make the genomic complementary construct G-ABCG14, a 4.1 kb genomic fragment was amplified by primers ABCG14-P9 and ABCG14-P10. The amplified fragment was digested by EcoRI and ligated to the EcoRI sites of pZP211 to form the G-ABCG14 construct. The AtABCG14 promoter was amplified by primers ABCG14-P11 and ABCG14-P12. The promoter region was then cloned into the pDONR207 entry vector via the BP reaction, designated pDONR207-pABCG14. To make the ABCG14::GUS and ABCG14::EGFP constructs, the promoter region of ABCG14 in pDONR207-pABCG14 was ligated into pMDC163 and pMDC107, respectively, via LR reactions. All the constructs described above were confirmed by sequencing. Hormone treatments Hormone treatments followed the method of Inoue et al. [36] with minor modifications. Briefly, seeds of selected genotypes were sown on half-strength MS medium containing BA, t Z, ACC or NAA with various concentrations. After chilling for 3 days, the plates were vertically incubated at 23 °C for 8 days and their root lengths in digital images were measured by Image J software (1.43). We calculated the relative root lengths by comparison with those of corresponding seedlings grown in hormone-free medium. The data presented are the mean of measurements from at least 12 plants. Determination of subcellular localization of ABCG14 Protoplasts isolated from young leaves of Arabidopsis plants grown under a 14 h light/10 h dark regime were transformed with column-purified plasmid DNA as previously described [42] . After 24-h incubation in the dark, the protoplasts were analysed for the presence of green fluorescence. 10-DAG transgenic seedlings harbouring 35S::EGFP-ABCG14 were used for protein localization. Cotyledon leaves and the first pair of true leaves were stained with 1 μg ml −1 PI (Sigma-Aldrich) or 10 μM FM4-64 (Molecular Probes) for 10~30 min. Cells in the leaves were also plasmolysed in 30% sucrose solution for about 1 h before staining in PI or FM4-64 in a 30% sucrose solution. Images were captured using a Leica DMI6000 microscope. GFP was detected using a 488-nm laser with a 505–530 nm filter. PI and FM4-64 staining were detected using a 488-nm laser with a 600–650 nm filter. Images were processed by Adobe Photoshop 8.0 (Adobe Systems, Mountain View, CA). Membrane preparation and gel-blot analysis Microsome preparation was followed by the procedure described in Miao and Liu [43] . Briefly, Arabidopsis seedlings (12-DAG) harboring 35S::EGFP-AtABCG14 expression cassette were ground with 50 mM Tris buffer A (pH 8.0) containing 2 mM EDTA, 20% Glycerol, 1 mM DTT and a 1X Protease inhibitor cocktail (PIC). The homogenate was filtered through Miracloth and centrifuged twice at 5,000 g for 15 min to remove the debris. Supernatants were centrifuged at 100,000 g for 1 h to pellet the microsomal membranes. The resulting microsomes were resuspended in 5 mM potassium phosphate buffer B (pH 7.8) containing 330 mM sucrose, 5 mM KCl, 1 mM DTT and 0.1 mM EDTA and 1X PIC. The plasma membranes were purified further from the microsomal preparation by partitioning in an aqueous-polymer two-phase system according to Larsson et al. [32] Briefly, the final weight of 9 g microsomal preparation in buffer B was added to 27 g of buffer C containing 5 mM potassium phosphate (pH 7.8), 330 mM sucrose, 5 mM KCL, 1 mM DTT, 0.1 mM EDTA, 1X PIC, 8.6% (w/w) Dextran T500 and 8.6% (w/w) polyethylene glycol 3,350, then mixed and partitioned by about 50 inversions. The two phases were separated by spinning at 1,500 g for 4 min. The resulting upper and lower phases were diluted using buffer B (pH 7.8) for three times and ten times, respectively, and centrifuged at 100,000 g for 2 h to obtain the membrane pellets. All procedures above were performed at 4 °C. The two-phase pellets as well as total microsomes were resuspended in 1X SDS buffer, heated at 70 °C for 10 min and developed on 10% SDS–PAGE gel. Immunoblots were probed with antibodies against GFP (Invitrogen A6455), Arabidopsis plasma membrane H + -ATPase (Agrisera AS07-260), vacuolar H + -pyrophosphatase (Operon Biotechnologies COP-080001), according to the standard procedure of gel blot. The cropped and full immunobloting images are presented in Fig. 4 and Supplementary Fig. 10 , respectively. Gene expression analysis Total RNA was prepared from Arabidopsis flower tissues using Trizol reagent (Invitrogen). To remove any contaminating DNA, the samples were treated with DNase (RNase-free DNase Kit; Promega). The reverse transcriptional reaction was performed using M-MLV Reverse Transcriptase (Promega). Quantitative PCR was undertaken using a MyIQ-Cycler (Bio-Rad) and IQ SYBR Green Supermix (New England Biolab) according to the manufacturer’s instructions with the following cycles: 10 min at 95 °C, followed by 40 cycles of 15 s at 95 °C, 25 s at 58 °C and a final extension of 40 s at 72 °C. The gene-specific primers ABCG14-P1 and ABCG14-P2 were used in RT–PCR to amplify the AtABCG14 gene, in which the ACTIN 2 gene was amplified by primers Actin 2F and Actin 2R as the control. For qRT–PCR, the AtABCG14 gene-specific primers ABCG14-P13 and ABCG14-P14 were used, the ACTIN 2 gene amplified with Actin 2QF and Actin 2QR or UBIQUITIN 10 gene amplified with Ub10F and Ub10R primers was used for quantitative normalization. The expression level of AtABCG14 , after normalization to that of ACTIN 2 or UBIQUITIN 10 control gene, is expressed as the relative value to the highest level in root tissue (in Fig. 3k ) or to the level in wild-type seedlings ( Figs 5f and 6a ) that was expressed as a value of 1. GUS staining and light microscopy Histochemical analysis of the GUS reporter enzyme was performed according to Jefferson et al. [44] with minor modifications. Briefly, tissues from transgenic plants were collected in glass vials containing ice-cold 90% acetone and incubated for 30 min at room temperature, then transferred into the reaction buffer and incubated for 1 to 12 h at 37 °C. After staining, pigments in the samples were destained with 70% ethanol, and the GUS staining pattern was recorded with a digital camera (Nikon DC3000) or a microscope (Leica DM5500B). For sectioning, plant tissues were fixed with formalin-acetic acid-alcohol (1.8% formalin, 5% acetic acid and 90% methanol) and embedded in paraffin; 8-μm thick sections were cut. Cytokinin profiling Arabidopsis seeds of selected genotypes were grown on half-strength MS medium supplemented with 3% sucrose. 10-DAG seedlings were used for cytokinin profiling. The roots and shoots of the seedlings were separated carefully with a razor at the junction between roots and hypocotyls. Approximately 20 mg fresh roots or shoots were freeze-dried in a microtube with a screw cap. The cytokinin extraction and profiling essentially followed a previously described method [28] . Briefly, the plant materials in 2.0 ml micro-centrifuge were mixed with the following stable isotope-labelled cytokinin internal standards at a concentration of 0.5 pmol of each compound per 50 μl of Bieleski buffer: [ 13 C 5 ] c Z, [ 13 C 5 ] t Z, [ 2 H 5 ] t ZR, [ 2 H 5 ] t Z7G, [ 2 H 5 ] t Z9G, [ 2 H 5 ] t ZOG, [ 2 H 5 ] t ZROG, [ 2 H 5 ] t ZMP, [ 2 H 3 ]DHZ, [ 2 H 3 ]DHZR, [ 2 H 3 ]DHZ9G, [ 2 H 7 ]DHZOG, [ 2 H 3 ]DHZMP, [ 2 H 6 ]iP, [ 2 H 6 ]iPR, [ 2 H 6 ]iP7G, [ 2 H 6 ]iP9G and [ 2 H 6 ]iPMP. They then were extracted in Bieleski solvent using a MM 301 vibration mill (Retsch GmbH & Co. KG, Haan, Germany). The tube’s contents were ultrasonicated and then incubated for 30 min at 4 °C. After centrifugation, the supernatants were transferred onto StageTips and purified according to the protocol described in Svacinova et al. [28] After elution, we collected the eluates and evaporated them to dryness in a Speed-Vac concentrator RC1010 (Jouan, Winchester, UK). Thereafter, we dissolved them in 20 μl of 10% methanol, and 10 μl of each sample was injected on to a reversed-phase column (Acquity UPLCW BEH C18, 1.7 μm, 2.1 mm × 150 mm, Waters). The samples were eluted in a 24-min gradient composed of methanol (A) and 15 mM ammonium formate pH 4.0 (B) at a flow rate of 0.25 ml min −1 , with a binary gradient: 0 min, 5:95 (A:B), 7.0-min isocratic elution, 5:95 (A:B), 9.0-min linear gradient, 20:80 (A:B), 7.0-min linear gradient, 50:50 (A:B) and 1 min isocratic elution, 50:50 (A:B). The effluent was passed through an ultraviolet-diode array detector and the tandem mass spectrometer Xevo TQ MS without post-column splitting. The parameter settings were followed as described previously [28] . We quantified them using a standard isotope-dilution method. We determined the ratio of endogenous cytokinin to the appropriate labelled standard and further quantified the level of endogenous compounds in the original extract, according to a known quantity of an added internal standard. Cytokinin tracer-uptake assay Arabidopsis seeds of selected genotypes were grown on half-strength MS medium supplemented with 3% sucrose. 10~12-DAG seedlings were used for the in planta isotope feeding. For root-feeding experiments, the root tips of atabcg14 mutants, the complementary line harbouring AtABCG14::EGFP-AtABCG14 and wild-type seedlings were immersed in 5 mM MES-KOH (pH 5.6) buffer containing C 14 - t Z (American Radiolabeled Chemicals, 3,700 Bq ml −1 , final concentration 5 nM) or S-adenosyl- L -C 14 -methionine (American Radiolabeled Chemicals, 3,700 Bq ml −1 , final concentration 5 nM) as a control. After 4 h, the roots and shoots of the seedlings were carefully separated using a razor at the junction between roots and hypocotyls. The shoots and roots from three seedlings of each genotype were pooled (separately) as replicates. The roots were washed again with 1 ml 5 mM MES-KOH (pH 5.6) buffer three times. For the time–course feeding experiment, the root tips of both wild-type and mutant seedlings were incubated with 5 nM C 14 - t Z in 5 mM MES-KOH (pH 5.6) buffer for 0.5, 1, 2, 3 and 5 h, and the shoots of seedlings were collected. The seedling samples were then mixed with 200 μl bleach and incubated at 55 °C for 2 h to solubilize the tissues. Radioactivity was quantified by a scintillation counter. For stable C 13 - t Z feeding, 12-DAG wild-type and mutant seedlings were incubated with 5 nM stable labelled chemical in 5 mM MES-KOH (pH 5.6) buffer for 4 h. The roots and shoots from 4~6 seedlings were separated, weighed and freeze-dried in a microtube with a screw cap for processing their extraction and analysis by LC-MS [28] . To feed C 14 - t Z or -SAM into the detached leaves, cotyledon leaves and the first pair of true leaves from three to five 10~12-DAG seedlings of the wild type and overexpression line harbouring 35S::GFP-AtABCG14 were weighed, then incubated in 150 μl of the feeding buffer containing C 14 - t Z or -SAM as described above. After 1 h incubation, the feeding solution was removed and the leaves were washed three times with 1 ml 5 mM MES-KOH (pH 5.6) buffer. For our time–course experiments, the fed leaves were sampled after an incubation of 5, 15, 30, 45 or 60 min. For sodium vanadate treatment, the sampled leaves were pre-treated in 150 μl 5 mM MES-KOH (pH 5.6) buffer with 1 mM sodium vanadata for 30 min, then the buffer was replaced with 150 μl 5 mM MES-KOH (pH 5.6) buffer containing 1 mM sodium vanadata and 5 nM C 14 - t Z and incubated for 1 h. After collecting and washing, the leaf samples were mixed with 200 μl bleach and incubated at 55 °C for 2 h to solubilize the tissue. Radioactivity was quantified by a scintillation counter. How to cite this article: Zhang, K. et al. Arabidopsis ABCG14 protein controls the acropetal translocation of root-synthesized cytokinins. Nat. Commun. 5:3274 doi: 10.1038/ncomms4274 (2014).